Enhancement of biological reactions on cell surfaces via macromolecular crowding The reaction of macromolecules such as enzymes and antibodies with cell surfaces is often an inefficient process, requiring large amounts of expensive reagent. Here we report a general method based on macromolecular crowding with a range of neutral polymers to enhance such reactions, using red blood cells (RBCs) as a model system. Rates of conversion of type A and B red blood cells to universal O type by removal of antigenic carbohydrates with selective glycosidases are increased up to 400-fold in the presence of crowders. Similar enhancements are seen for antibody binding. We further explore the factors underlying these enhancements using confocal microscopy and fluorescent recovery after bleaching (FRAP) techniques with various fluorescent protein fusion partners. Increased cell-surface concentration due to volume exclusion, along with two-dimensionally confined diffusion of enzymes close to the cell surface, appear to be the major contributing factors. Cell-surface engineering has been increasingly explored as a means of enhancing in vivo cell survival and function [1] , [2] , [3] . For instance, stem cells have been modified to enhance homing [1] , T and B cells have been modified for targeted delivery of therapeutics to tumours [3] , tPA-carrying red blood cells (RBCs) have been generated for selective dissolution of nascent clots [4] , enzymatically modified RBCs have been produced as universal donor RBCs [5] , [6] and polymer conjugation of RBCs and tissues camouflaged their surface antigens from immune system recognition and destruction [7] , [8] , [9] . Although there is tremendous potential for cell-surface modification with macromolecular agents (enzymes, polymers and proteins) in many practical applications, the generally poor association of macromolecules with cell surfaces (~0.5%) [7] due to the repulsion of two hydrophilic entities requires high concentrations of reagent, making the process costly. Further, attempts to use excess cell-surface reactive macromolecules to drive the process are often harmful to cells. Thus, the development of a general process or method that could enhance biological reactions on cell surfaces without damaging the cells or requiring modified reagents could be of considerable value by lowering costs of cell-surface engineering technologies and thereby enhancing their commercial potential. Most of the biological processes in cells occur in crowded conditions, with biopolymer concentrations within the cells ranging from 100 to 400 mg ml −1 (refs 10 , 11 , 12 ). Crowding a system with neutral macromolecules favours associations that result in net reduction of excluded volume, thus altering the reaction rates and association constants of biological reactions [13] , [14] , [15] , [16] , [17] , [18] , [19] , and the effects can be highly nonlinear if macromolecules themselves are involved in the process [20] . Crowding has been used to impact the outcome of biological and biotechnological processes [16] , [17] , [18] , [19] , [20] , [21] , [22] , [23] , [24] , [25] , [26] , [27] , [28] , [29] , [30] , [31] , [32] , [33] . However, most of the information currently available on macromolecular crowding focuses on experiments performed in solution conditions. Very little is known about reactions on surface-associated structures or cell surfaces. Although the reaction rates on the cell surface in crowded conditions are theoretically predicted to be higher [14] , [15] , this has not been proven experimentally and no practical application has been reported so far for enhanced surface events based on macromolecular crowding. The ABO blood group antigens, discovered by Landsteiner [34] , are the most potent antigens to be considered in blood transfusion and are present at ~10 6 antigens per cell [35] . The antigenicity of ABO blood groups is defined by the structures of the carbohydrate unit(s) at the outer termini of glycoproteins and lipids on the surface of RBCs [36] , [37] as illustrated in Fig. 1a . A common H antigen (in O type) is decorated with α-galactose in B-type or α- N -acetylgalactosamine in A type; thus, A- and B-type blood immunoreact with each other and with AB. However, blood from O blood group individuals can be transfused to persons with any other blood group and is considered to be the universal donor blood [5] . There has always been a demand for O − group blood in hospitals around the world to deal with emergency trauma situations, pediatric transfusions, shortage of blood from other donor groups and cases of lack of clarity of patient blood group [5] , [6] . To overcome this shortage and to enhance the safety of blood transfusions, the enzymatic conversion of A, B or AB blood groups to the universal donor O group blood by the use of glycosidases to remove the Gal or GalNAc residues has emerged as a useful strategy [6] . However, the biggest obstacle to the widespread use of enzymatic approaches for removal of blood group antigens has been the inefficiency of the enzymes used. Consequently, large quantities of enzymes are needed for complete antigen cleavage and this excess enzyme must then be thoroughly removed from the modified cells after treatment [6] , [38] . 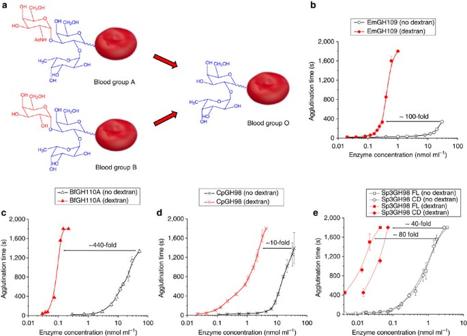Figure 1: Influence of macromolecular crowding on the activity of enzymes working on the red blood cell surface. (a) Structures of AB antigenic carbohydrates on RBC surface and their conversion to O blood group. The hydrolase activity of (b) EmGH109 (α-N-acetyl-galactosaminidase fromE. miricola), (c) BfGH110A (α-galactosidase fromB. fragilis), (d) CpGH98 (family 98 endoglycosidase fromC. perfringens), and (e) Sp3GH98 FL and Sp3GH98 CD (full length and catalytic domain of family 98 endoglycosidase fromS. pneumoniaSP3-BS71) enzymes on RBCs in the absence and presence of macromolecular crowder dextran 40 kDa at 300 mg ml−1concentration. EmGH109 is an ‘A’ blood group cleaving enzyme; all other enzymes cleave ‘B’ blood group antigens. FL stands for full-length enzyme with carbohydrate binding domain attached. CD stands for catalytic domain. The removal of blood group carbohydrate antigens from the cell surface is measured from the haemagglutination time of enzymatically treated RBCs on treatment with corresponding monoclonal antibodies. RBCs (10% haematocrit) were treated with different concentrations of enzymes for 1 h at room temperature (22 °C) in the absence and presence of dextran 40 kDa (300 mg ml−1) in PBS buffer at pH 7.4. See alsoSupplementary Figs 1–3. Data points represent the average of three experimental measurements and the error bars are the s.d. around the mean. Figure 1: Influence of macromolecular crowding on the activity of enzymes working on the red blood cell surface. ( a ) Structures of AB antigenic carbohydrates on RBC surface and their conversion to O blood group. The hydrolase activity of ( b ) EmGH109 (α- N -acetyl-galactosaminidase from E. miricola ), ( c ) BfGH110A (α-galactosidase from B. fragilis ), ( d ) CpGH98 (family 98 endoglycosidase from C. perfringens ), and ( e ) Sp3GH98 FL and Sp3GH98 CD (full length and catalytic domain of family 98 endoglycosidase from S. pneumonia SP3-BS71) enzymes on RBCs in the absence and presence of macromolecular crowder dextran 40 kDa at 300 mg ml −1 concentration. EmGH109 is an ‘A’ blood group cleaving enzyme; all other enzymes cleave ‘B’ blood group antigens. FL stands for full-length enzyme with carbohydrate binding domain attached. CD stands for catalytic domain. The removal of blood group carbohydrate antigens from the cell surface is measured from the haemagglutination time of enzymatically treated RBCs on treatment with corresponding monoclonal antibodies. RBCs (10% haematocrit) were treated with different concentrations of enzymes for 1 h at room temperature (22 °C) in the absence and presence of dextran 40 kDa (300 mg ml −1 ) in PBS buffer at pH 7.4. See also Supplementary Figs 1–3 . Data points represent the average of three experimental measurements and the error bars are the s.d. around the mean. Full size image Here we report the development of a facile method to enhance these cell-surface reactions based on macromolecular crowding. Using this approach, we have shown that the activities of glycosidases working on the cell surface can be increased over 440-fold. The mechanism of enhancement of enzymatic activity on the cell surface has been studied by investigating the deposition, mobility and exchange of enzyme on the cell surface by confocal microscopy analysis and fluorescent recovery after photobleaching (FRAP) techniques. We have also shown that this crowding method can be applied to other cell-surface reactions involving macromolecules. The approach therefore has great potential to reduce costs of production of not only universal RBCs but also any product in which a cell surface is modified using a macromolecular reagent. Choice of cell-surface active enzymes We tested the macromolecular crowding effect on a number of enzymes that are active on cell-surface oligosaccharides. Useful α- N -acetylgalactosaminidases and α-galactosidases were identified from glycoside hydrolase (GH) family 109 and 110 enzymes, respectively, in an earlier screen [6] . The GH109 enzyme from Elizabethkingia miricola (EmGH109) is active on A blood group antigens, cleaving the terminal N -acetylgalactosamine from the oligosaccharide antigen, whereas the GH110 enzyme from Bacteriodes fragilis (BfGH110A) operates on B blood group antigens, cleaving the terminal galactose. Certain members of the GH family GH98 also cleave A and B blood group antigens, but in this case are endo-β-galactosidases, cutting off the entire trisaccharide [39] . The GH98 enzymes from Clostridium perfringens (CpGH98) and from Streptococcus pneumoniae SP3-BS71 (Sp3GH98) work on both A and B blood group antigens, cleaving a Galβ1-4GlcNAc linkage between the terminal trisaccharide antigenic determinant and the core oligosaccharide attached to the cell surface [39] , [40] . The version of CpGH98 containing only the catalytic domain was studied, while both the full-length S. pneumonia enzyme (Sp3GH98 FL) containing carbohydrate binding domains and the catalytic domain (Sp3GH98 CD) alone were tested. Influence of crowder on cell-surface glycosidase activity We initially investigated the glycosidase activity of the five different blood group cleaving enzymes in the absence and presence of a neutral macromolecular crowder, 40 kDa dextran (300 mg ml −1 ) [16] , [22] , at physiological pH ( Fig. 1 ). The removal of cell-surface carbohydrate antigens was assessed by measuring the time after enzymatic treatment at which RBCs aggregate in the presence of blood group-specific antibodies: the haemagglutination time ( Fig. 1 and Supplementary Fig. 1A,B ). A longer agglutination time correlates with more effective enzymatic removal of antigens, with no haemagglutination within 30 min being considered complete removal of blood group antigens, as confirmed by other methods (see below). As shown in Fig. 1 , the addition of a crowder dramatically enhanced the enzymatic activities in all cases, with substantially less enzyme being required to achieve similar levels of blood group antigen removal to that needed in the absence of the crowder ( Fig. 1b–e ). As shown, enhancement factors varied by enzyme from 10-fold to 440-fold, allowing full antigen removal at very low enzyme levels in some cases. Interestingly, the presence of a carbohydrate binding domain had no beneficial effect in the absence of crowder, but does in the presence of crowder. This enhancement in antigen cleavage was further evaluated using Food and Drug Administration (FDA)-approved blood phenotyping Micro Typing System cards (MTS cards), as shown in Supplementary Fig. 1C–E . Antibodies immobilized on the column agglutinate RBCs bearing that antigen, which then do not penetrate the mini gel on centrifugation (see, for example, Supplementary Fig. 1D : score 4+). Complete blood group antigen removal is indicated by the migration of RBCs to the bottom of the gel (score 0). As seen in Supplementary Fig. 1C , representative MTS card analysis of blood group ‘A’ RBCs treated with amounts of EmGH109 in the range from 1 to 30 nmol ml −1 in the absence of the crowder give a score of 4+ to 3+ indicative of relatively little removal of ‘A’ group antigen from the cell surface ( Supplementary Fig. 1C ). However, the inclusion of dextran in the enzymatic reactions resulted in complete removal of ‘A’ group antigens from the cell surface even at the lowest EmGH109 concentration of 1 nmol ml −1 (score ‘0’) ( Supplementary Fig. 1C ). Similar results were obtained for removal of B antigens using the enzymes Sp3GH98 CD and Sp3GH98 FL ( Supplementary Fig. 1D,E ), confirming the potential of macromolecular crowding in enhancing the activity of different glycosidases on the RBC surface. The removal of cell-surface antigens by glycosidases was further probed using flow cytometry analysis. In these experiments, blood group ‘A’ antigen-cleaving enzyme, EmGH109, was used along with a fluorescently labelled monoclonal ‘A’ antibody. As shown in Supplementary Fig. 1F , using a concentration of 30 nmol ml −1 , only partial removal of blood group A antigens was observed. By contrast, in the presence of dextran only 1 nmol ml −1 of EmGH109 was needed for quantitative removal of ‘A’ antigens, as was also seen by MTS card analysis. The enzymatic removal of carbohydrate antigens was further probed by optical microscopy ( Supplementary Fig. 1G–K ) using Sp3GH98 FL enzyme and blood group ‘B’ antibody. Control and enzyme-treated RBCs were incubated with antibody and visualized under a microscope. Cells aggregate in the presence of antibodies when antigens have not been fully removed. Again, the inclusion of dextran resulted in removal of cell-surface carbohydrate antigens using only very small amounts of enzyme, as indicated by the absence of RBC aggregation. Similar results were obtained for the other enzymes. This use of three different methods confirms that antigen removal is indeed being achieved. Impact of crowder structure on cell-surface activity Having demonstrated the phenomenon with dextran, we next investigated the effectiveness of other water-soluble neutral polymers, to optimize conditions. Samples of ficoll, hyperbranched polyglycerol (HPG), polyethylene glycol (PEG) and polyvinylpyrrolidone (PVP) of varying molecular weight were studied. The concentrations of polymers used mimic biopolymer concentrations in living systems: ~50 mg ml −1 in the interstitial fluids [11] , ~100 mg ml −1 in blood plasma [10] and ~300 mg ml −1 in the cell interior [12] . Polymers were first screened for induction of hemolysis or cell aggregation, and both PEG and PVP were found to fail this test, as shown ( Supplementary Fig. 2A–C ). However, dextran, ficoll and HPG induced no cell aggregation or hemolysis ( Supplementary Fig. 2D–G ), and so were selected for further study. The influence of these latter crowders on the enzymatic cleavage of blood group antigens is given in Fig. 2 (for Sp3GH98 FL (at constant 0.013 nmol ml −1 )) and in Supplementary Fig. 3 (for Sp3GH98 CD (at constant 0.043 nmol ml −1 )). The number of RBCs (10% haematocrit) used was kept constant and haemagglutination time was measured before and after enzyme treatment. Cell-surface enzymatic activity increased with crowder concentration, irrespective of the molecular weight or type of crowder used. However, a smaller activity enhancement was observed at lower crowder concentrations (50 and 100 mg ml −1 ) than at higher levels (300 mg ml −1 ). The molecular weight of the crowder seems to have only a minor role and the effect is only visible at higher concentrations (300 mg ml −1 ). HPG works more efficiently as a crowder than do dextran and ficoll for Sp3GH98 FL at all molecular weights ( Fig. 2c ) and all concentrations ( Fig. 2d ), and is comparable to dextran for Sp3GH98 CD ( Supplementary Fig. 3 ). 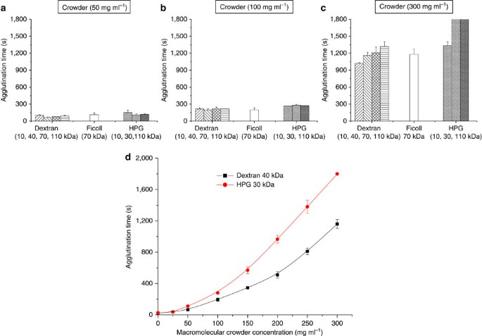Figure 2: The impact of the structure, molecular weight and concentration of macromolecular crowder on the enzymatic activity. The effect of different macromolecular crowders and their molecular weights on the hydrolytic activity of Sp3GH98 FL (at constant a concentration of 0.013 nmol ml−1) on blood group B RBCs at (a) 50 (b) 100 and (c) 300 mg ml−1concentration. These values reflect the concentration of macromolecules in interstitial fluids, blood plasma and the cell interior, respectively. The extent of removal of blood group B carbohydrate antigens is evaluated from RBC agglutination time after treatment with murine anti-human B monoclonal antibody. RBCs (10% haematocrit) were treated with Sp3GH98 FL (at constant 0.013 nmol ml−1) at room temperature (22 °C) for 1 h in the absence and presence of different crowders (dextran, ficoll and HPG) at three concentrations. Different molecular weights of dextran (10, 40, 70 and 110 kDa), ficoll (70 kDa) and HPG (10, 30 and 110 kDa) were used. (d) The impact of macromolecular crowder dextran (40 kDa) and HPG (30 kDa) concentration on hydrolytic activity of Sp3GH98 FL (0.013 nmol ml−1) on RBCs. Enzyme-treated RBCs were incubated with murine anti-human B monoclonal antibody and the haemagglutination time measured. Data points represent the average of three experimental measurements and the error bars are the s.d. around the mean. Figure 2: The impact of the structure, molecular weight and concentration of macromolecular crowder on the enzymatic activity. The effect of different macromolecular crowders and their molecular weights on the hydrolytic activity of Sp3GH98 FL (at constant a concentration of 0.013 nmol ml −1 ) on blood group B RBCs at ( a ) 50 ( b ) 100 and ( c ) 300 mg ml −1 concentration. These values reflect the concentration of macromolecules in interstitial fluids, blood plasma and the cell interior, respectively. The extent of removal of blood group B carbohydrate antigens is evaluated from RBC agglutination time after treatment with murine anti-human B monoclonal antibody. RBCs (10% haematocrit) were treated with Sp3GH98 FL (at constant 0.013 nmol ml −1 ) at room temperature (22 °C) for 1 h in the absence and presence of different crowders (dextran, ficoll and HPG) at three concentrations. Different molecular weights of dextran (10, 40, 70 and 110 kDa), ficoll (70 kDa) and HPG (10, 30 and 110 kDa) were used. ( d ) The impact of macromolecular crowder dextran (40 kDa) and HPG (30 kDa) concentration on hydrolytic activity of Sp3GH98 FL (0.013 nmol ml −1 ) on RBCs. Enzyme-treated RBCs were incubated with murine anti-human B monoclonal antibody and the haemagglutination time measured. Data points represent the average of three experimental measurements and the error bars are the s.d. around the mean. Full size image As macromolecular associations in crowded conditions are influenced by the volume excluded by background molecules [16] (hydrated neutral polymers in this case), the amount of free water in the system was measured from the fusion enthalpy of free water by differential scanning calorimetry ( Supplementary Fig. 4 ). The amount of free water, which represents the volume available for enzyme in the system, decreased with increase in crowder concentration. This increase in volume exclusion correlates with increased cell-surface enzymatic activity at higher crowder concentrations, as seen in ( Fig. 2c,d ). Mechanism of enhancement To probe the underlying mechanism of enzymatic activity enhancement on the cell surface, we investigated the effect of crowders on the enzymatic cleavage of small molecule substrates in solution, the concentration of the enzyme on the cell surface, the diffusion/mobility of the enzyme on the cell surface and the exchange of enzymes in solution with enzymes on the cell surface. Enzymatic cleavage of small molecule substrates To confirm that the effects of crowders were not due to inherent effects on the reactivity of the enzyme, we measured kinetic parameters for cleavage of small molecule substrates, in the absence and presence of crowders, by two enzymes, CpGH98 and BfGH110A. As shown in Supplementary Table 1 , the inclusion of polymer resulted in no change in either k cat or K m for either enzyme relative to buffer alone. Concentration of enzymes on the cell surface For these experiments, RBCs were immobilized on a glass substrate and a green fluorescent protein (GFP)-labelled, catalytically inactive mutant version of the enzyme (GFP-Sp3GH98 E558A CD) was used. A representative scheme for the RBC immobilization and the confocal microscopy measurements is shown in ( Supplementary Fig. 5A ). At a constant GFP-Sp3GH98 E558A CD concentration, the fluorescence intensity on the cell surface will correlate with the concentration of enzyme on the surface. Representative images in PBS, dextran (90 mg ml −1 ) and dextran (320 mg ml −1 ) are shown in Fig. 3a , and these clearly show that fluorescence intensity on the cell surface increases dramatically with increasing concentration of the macromolecular crowder (see also Supplementary Fig. 5B,C ). The normalized fluorescence intensity values shown in Fig. 3b indicate a ~5.5-fold increase in enzyme concentration on the cell surface compared with that in PBS at the maximum concentration of dextran studied. A control experiment with immobilized enzyme on the glass surface (without cells) showed no changes in fluorescent intensity with dextran concentration ( Supplementary Fig. 5D–F ), indicating that the increased fluorescence intensity observed on the cell surface with dextran ( Fig. 3a,b ) is due to the higher concentration of enzyme on the cell surface and not due to some solvation effect. 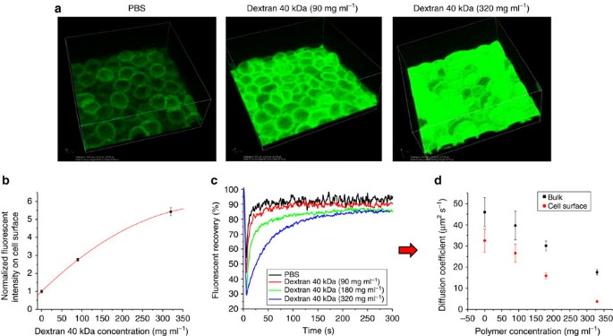Figure 3: Influence of macromolecular crowding on cell-surface enzyme concentration and mobility of C-terminally tagged GFP-labelled (GFP-Sp3GH98 E558A CD, green) mutant enzyme. RBCs were immobilized initially onto a glass surface using poly(L-lysine) and glutaraldehyde (see alsoSupplementary Fig. 5a). To surface-attached RBCs, a solution containing GFP-Sp3GH98 E558A CD (1.3 nmol ml−1) supplemented with different concentrations of dextran 40 kDa in PBS buffer (pH 7.4) was added. Fluorescence on the cell surface was monitored using a Nikon C2+ Eclipse Ti-E confocal microscope 10 min after the addition of enzyme to the cells (see alsoSupplementary Fig. 5). (a) Representative three-dimensional images of cells obtained by confocal microscopy at × 60 oil immersion objective using 90 and 320 mg ml−1dextran concentrations. The image size is 50 × 50 × 20 μm. (b) Normalized intensity of GFP-labelled Sp3GH98 E558A CD on cell surface at different crowding conditions. The values were obtained by measuring the fluorescence intensity at three randomly chosen spots (5,000 μm2area) on the cell surface in a representative experiment. The error bars are the s.d. around the mean. The experiment was repeated with three different donors giving similar results. (c) The diffusion of GFP-Sp3GH98 E558A CD in bulk and on the cell surface measured using the technique of FRAP in the absence and presence of macromolecular crowder dextran at different concentrations (90, 180 and 320 mg ml−1). Representative results of the fluorescence recovery of GFP-Sp3GH98 E558A CD on the cell surface after bleaching is shown. Experimental conditions were similar to that ofa. (d) Diffusion coefficients of GFP-labelled Sp3GH98 E558A CD both in bulk solution and on the cell surface were obtained using a procedure developed by Axelrod D.et al.38, as detailed in the experimental section. Data points represent the average of three experimental measurements and the error bars are the s.d. around the mean. Figure 3: Influence of macromolecular crowding on cell-surface enzyme concentration and mobility of C-terminally tagged GFP-labelled (GFP-Sp3GH98 E558A CD, green) mutant enzyme. RBCs were immobilized initially onto a glass surface using poly( L -lysine) and glutaraldehyde (see also Supplementary Fig. 5a ). To surface-attached RBCs, a solution containing GFP-Sp3GH98 E558A CD (1.3 nmol ml −1 ) supplemented with different concentrations of dextran 40 kDa in PBS buffer (pH 7.4) was added. Fluorescence on the cell surface was monitored using a Nikon C2+ Eclipse Ti-E confocal microscope 10 min after the addition of enzyme to the cells (see also Supplementary Fig. 5 ). ( a ) Representative three-dimensional images of cells obtained by confocal microscopy at × 60 oil immersion objective using 90 and 320 mg ml −1 dextran concentrations. The image size is 50 × 50 × 20 μm. ( b ) Normalized intensity of GFP-labelled Sp3GH98 E558A CD on cell surface at different crowding conditions. The values were obtained by measuring the fluorescence intensity at three randomly chosen spots (5,000 μm 2 area) on the cell surface in a representative experiment. The error bars are the s.d. around the mean. The experiment was repeated with three different donors giving similar results. ( c ) The diffusion of GFP-Sp3GH98 E558A CD in bulk and on the cell surface measured using the technique of FRAP in the absence and presence of macromolecular crowder dextran at different concentrations (90, 180 and 320 mg ml −1 ). Representative results of the fluorescence recovery of GFP-Sp3GH98 E558A CD on the cell surface after bleaching is shown. Experimental conditions were similar to that of a . ( d ) Diffusion coefficients of GFP-labelled Sp3GH98 E558A CD both in bulk solution and on the cell surface were obtained using a procedure developed by Axelrod D. et al . [38] , as detailed in the experimental section. Data points represent the average of three experimental measurements and the error bars are the s.d. around the mean. Full size image Mobility of enzymes on the cell surface The diffusion of GFP-Sp3GH98 E558A CD both in bulk and on the cell surface was measured using the technique of FRAP [41] , [42] , [43] , [44] , in which the fluorescence of a circular region on the cell surface is photobleached and the recovery of fluorescence due to in-migration of non-bleached enzyme is monitored ( Supplementary Movie 1 ). The FRAP recovery was measured in PBS and at different concentrations of 40 kDa dextran (90–320 mg ml −1 ). The FRAP recovery profile on the cell surface is shown in Fig. 3c and in the bulk medium (solution) in ( Supplementary Fig. 6A ). The diffusion coefficients of the GFP-Sp3GH98 E558A CD in solution and on the cell surface were calculated according to a method developed by Axelrod et al . [41] and values are given in Fig. 3d . The diffusion coefficient of GFP-Sp3GH98 E558A CD measured in solution in PBS (46±6.8 μm 2 s −1 ) correlates well with literature values for proteins such as fluorescein isothiocyanate (FITC)–streptavidin (50 μm 2 s −1 ) and FITC-BSA (68 μm 2 s −1 ) [45] . The diffusion rate of GFP-Sp3GH98 E558A CD in solution decreased with increase in concentration of dextran as expected; ~2.5-fold lower in the presence of 320 mg ml −1 dextran than in PBS alone. On the cell surface, the diffusion of GFP-Sp3GH98 E558A CD is slower than in bulk solution and the effects of dextran are greater, with diffusion constants dropping ~9-fold on addition of 320 mg ml −1 dextran to the PBS ( Fig. 3d ). Despite this slower surface diffusion, the majority (75±2%) of the surface-deposited enzyme is mobile in the presence of dextran (320 mg ml −1 ). This compares to 86±7% in bulk solution under similar conditions ( Supplementary Fig. 6B ), calculated from the fluorescence intensity of the bleached area before and after bleaching, and after recovery using equation (5) [46] . To confirm that fluorescence recovery on the cell surface is entirely due to translational diffusion and not to some other form of fluorescence recovery, the experiment was repeated with GFP-Sp3GH98 E558A CD immobilized on the cell surface by glutaraldehyde cross-linking, and indeed fluorescence recovery was seen to be abolished [47] , [48] ( Supplementary Movie 2 and Supplementary Fig. 6C ). Mechanism of surface exchange of enzymes It is not immediately obvious how the presence of a crowder could affect the lateral surface diffusion so greatly (ninefold). One possibility is that lateral diffusion is effected through a ‘hopping’ mechanism in which enzyme molecules dissociate, diffuse laterally in solution near the surface and then rebind. To probe this possibility, we constructed an additional fluorescent fusion protein with a cyan fluorescent protein (CFP-Sp3GH98 E558A CD) and used the pair of fluorescent fusion proteins of different colours to investigate possible exchange processes. Relative rates of surface association were first measured by placing a layer of PBS or crowder (transparent layer) on the cell surface, overlaying a layer of GFP-Sp3GH98 E558A CD and measuring the fluorescence on the cell surface as a function of time ( Fig. 4a–c ). Representative fluorescence images in PBS and in the presence of 40 kDa dextran at 180 and 320 mg ml −1 are shown ( Fig. 4b ). As expected, the diffusion of GFP-Sp3GH98 E558A CD to the cell surface is slower at higher crowder concentrations ( Fig. 4b,c ). 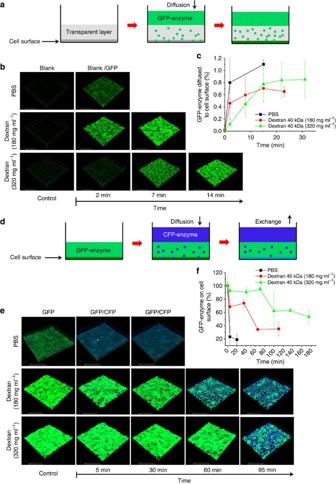Figure 4: Impact of crowding on cell-surface association and exchange of enzymes. C-terminally-tagged GFP-labelled-(GFP-Sp3GH98 E558A CD, green) and C-terminally tagged-CFP-labelled-(CFP-Sp3GH98 E558A CD, cyan) inactive mutant Sp3GH98 CD enzymes were used. (a) Experimental setup for the measurement of diffusion of enzymes to cell surface. A layer of PBS or crowder (transparent layer, 75 μl) with a minimal amount of GFP enzyme was added to RBCs. PBS or crowder (75 μl) that contained GFP enzyme (1.3 nmol ml−1) was then added and the fluorescence intensity on the cell surface was monitored with time. (b) Representative confocal images of cells covered with a transparent layer then overlaid with a GFP enzyme-containing layer incorporating different amounts of crowder at different time points. (c) Per cent of GFP enzyme on the cell surface in PBS at different concentrations of crowder at different time points. (d) Experimental setup for the measurement of exchange of enzymes to the cell surface. A layer of PBS or crowder (75 μl) that contains GFP enzyme (1.3 nmol ml−1) was added initially and allowed to equilibrate for 10 min, followed by the addition of 75 μl of CFP enzyme (10.7 nmol ml−1). (e) Representative confocal images of cells covered with a GFP-enzyme layer followed by a CFP-enzyme layer containing different amounts of crowder: the fluorescence intensity on the cell surface was followed with time using both the green and cyan channels at 488 and 457 nm, respectively. (f) Per cent of GFP enzyme present on cell surface after exchanging with CFP enzyme in the absence and presence of different amounts of crowder. Points incandfrepresent the average cell surface fluorescence intensity of three random areas (45,000 μm2), error bars are s.d. around the mean and lines simply provide guidance. The image sizes inbandeare around 80 × 80 × 10 μm. The per cent of GFP enzyme (~20%) present on cell surfaces in PBS after the exchange (equilibrium) process reflects the ratio of GFP/CFP enzymes added. A higher concentration of CFP enzyme was used for better visualization. Figure 4: Impact of crowding on cell-surface association and exchange of enzymes. C-terminally-tagged GFP-labelled-(GFP-Sp3GH98 E558A CD, green) and C-terminally tagged-CFP-labelled-(CFP-Sp3GH98 E558A CD, cyan) inactive mutant Sp3GH98 CD enzymes were used. ( a ) Experimental setup for the measurement of diffusion of enzymes to cell surface. A layer of PBS or crowder (transparent layer, 75 μl) with a minimal amount of GFP enzyme was added to RBCs. PBS or crowder (75 μl) that contained GFP enzyme (1.3 nmol ml −1 ) was then added and the fluorescence intensity on the cell surface was monitored with time. ( b ) Representative confocal images of cells covered with a transparent layer then overlaid with a GFP enzyme-containing layer incorporating different amounts of crowder at different time points. ( c ) Per cent of GFP enzyme on the cell surface in PBS at different concentrations of crowder at different time points. ( d ) Experimental setup for the measurement of exchange of enzymes to the cell surface. A layer of PBS or crowder (75 μl) that contains GFP enzyme (1.3 nmol ml −1 ) was added initially and allowed to equilibrate for 10 min, followed by the addition of 75 μl of CFP enzyme (10.7 nmol ml −1 ). ( e ) Representative confocal images of cells covered with a GFP-enzyme layer followed by a CFP-enzyme layer containing different amounts of crowder: the fluorescence intensity on the cell surface was followed with time using both the green and cyan channels at 488 and 457 nm, respectively. ( f ) Per cent of GFP enzyme present on cell surface after exchanging with CFP enzyme in the absence and presence of different amounts of crowder. Points in c and f represent the average cell surface fluorescence intensity of three random areas (45,000 μm 2 ), error bars are s.d. around the mean and lines simply provide guidance. The image sizes in b and e are around 80 × 80 × 10 μm. The per cent of GFP enzyme (~20%) present on cell surfaces in PBS after the exchange (equilibrium) process reflects the ratio of GFP/CFP enzymes added. A higher concentration of CFP enzyme was used for better visualization. Full size image To investigate the exchange of enzymes on the cell surface, GFP-labelled inactive mutant enzyme was first added to the cells under crowding (180 and 320 mg ml −1 dextran 40 kDa) and non-crowding conditions (PBS buffer) at 1.3 nmol ml −1 concentration. After equilibration, CFP-labelled inactive mutant enzyme was added to the solution at eightfold higher concentration (10.7 nmol ml −1 ) and the cell-surface fluorescence was monitored on green and cyan channels simultaneously ( Fig. 4d–f ). Representative fluorescence images for each condition at different time points are shown in Fig. 4e . As seen, in PBS the green fluorescence on the cell surface is rapidly replaced with blue reaching equilibrium, while in the presence of dextran this exchange occurs much more slowly, and in a dextran concentration-dependent manner ( Fig. 4e,f ). This exchange process was also observed by monitoring the green channel as seen in Supplementary Fig. 7 , where the fluorescence intensity on the cell surface decreased with time. This is completely consistent with the hopping model of lateral diffusion wherein the crowder primarily slows lateral diffusion within the solvent layer above the bound surface. Indeed, comparison of Figs 3d and 4f reveals that increasing the concentration of crowder from 180 to 320 mg ml −1 decreases rates of both diffusion and surface exchange by the same approximate threefold factor. It would therefore appear that a principal mechanism of rate enhancement involves a concentration of enzymes near the surface through molecular crowding such that when an enzyme releases from the surface it is largely confined within the surface layer and rebinds in preference to diffusing away ( Fig. 5 ). 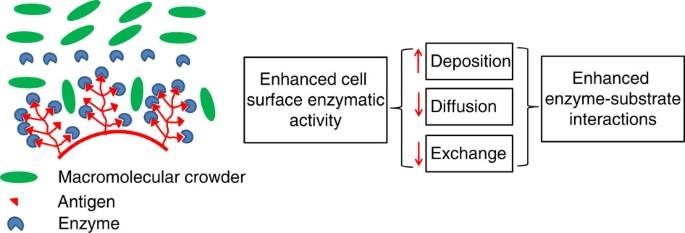Figure 5: Schematic representation of the proposed mechanism of enhancement of enzymatic activity on the cell surface under crowded conditions. A combination of increased surface concentration, decreased diffusion away and slow exchange of enzymes in the presence of macromolecular crowder is responsible for enhancing enzyme activity on cell surface. Other contributing factors include nature of the enzymes, possible changes in the glycocalyx and changes in accessibility to cell surface substrates in presence of crowders. Figure 5: Schematic representation of the proposed mechanism of enhancement of enzymatic activity on the cell surface under crowded conditions. A combination of increased surface concentration, decreased diffusion away and slow exchange of enzymes in the presence of macromolecular crowder is responsible for enhancing enzyme activity on cell surface. Other contributing factors include nature of the enzymes, possible changes in the glycocalyx and changes in accessibility to cell surface substrates in presence of crowders. Full size image Impact of crowding on other cell-surface reactions To investigate whether molecular crowding impacts cell-surface reactions other than the enzymatic removal of blood group antigens, the interactions of antibodies with cell-surface antigens and the removal of sialic acid from cell surfaces under crowded conditions were studied. As shown in Supplementary Fig. 8A,B , crowding significantly enhanced the interaction of all tested antibodies (fixed concentration) with the RBC surface: anti Rhesus D and anti CD 47 antibodies. For example, the binding of anti CD47 antibody to the RBC surface increased ~8-fold in the presence of 30 kDa HPG at 300 mg ml −1 compared with that in PBS buffer alone ( Supplementary Fig. 8A,B ). Among the crowders, HPG is a slightly better enhancer than ficoll for antibody-antigen binding ( Supplementary Fig. 8A,B ). Relative rates of neuraminidase-catalysed removal of sialic acid from RBC surfaces were investigated by measuring the electrophoretic mobility of treated RBCs [49] . A substantially greater decrease in electrophoretic mobility of RBCs exposed to neuraminidase under crowded conditions was observed compared with that in the absence of crowder, indicating a greater extent of sialic acid removal from the cell surface ( Supplementary Fig. 8C ). A major impediment to the application of macromolecule-based cell-surface engineering is the requirement for large amounts of reagents due to the low levels of their association with the cell surface. For example, the generation of universal donor RBCs via enzymatic cleavage of cell-surface antigens has languished in the early stages of clinical trials in large part due to the costs of producing the substantial amounts of enzymes required for the process. In this report, using relatively cheap, cell compatible neutral polymers such as dextran and ficoll as macromolecular crowders, we demonstrate a general method for enhancing cell-surface enzymatic activity. Several advantages accrue from this finding. First, the quantities of enzyme required for cell-surface modification can be considerably reduced. Thus, with the help of macromolecular crowding, A + , B + and AB + RBCs ( + indicates presence of Rh factor) have been converted to O + RBCs at physiological pH within an hour at room temperature using only a few μg ml −1 of EmGH109 and Sp3GH98 enzymes ( Table 1 and Supplementary Fig. 9A ). Similarly, B − RBCs ( − indicates absence of Rh factor) have been converted to O − cells. In the case of AB + cells, a combination of EmGH109 and Sp3GH98 CD enzymes was used to convert A and B antigens to O blood groups ( Table 1 and Supplementary Fig. 9A ). A simple calculation reveals that conversion of one unit of B-RBCs (200 ml packed RBCs) to universal donor RBCs requires only a few hundred micrograms of blood group B-cleaving Sp3GH98–FL enzyme in crowded conditions. A second advantage is that the process for cleaning the modified cells after enzymatic treatment will be much simpler due to the very small quantities of enzymes used, thereby helping minimize the risk of immunogenic reactions due to surface-adsorbed macromolecules [6] . Washing of the cells will remove both the highly water-soluble cell compatible polymers and the enzyme: indeed a washing procedure is already used in blood banks before the use of RBCs; thus, incorporation of this new rate-enhancement protocol will not be out of line with current blood bank practices [50] . Importantly, the treated cells under crowded conditions had normal physiochemical properties, as indicated from their normal structural and functional integrity ( Supplementary Figs 9B, 10 and 11 ) highlighting the potential clinical utility of the technique. This robustness is not surprising, as RBCs circulate under crowded conditions in the plasma at ~100 mg ml −1 and undergo repeated shape changes while passing through capillaries. This approach moves the concept of universal blood closer to an economic reality. We anticipate that this general approach of enhanced cell surface reactions can be translated to other types of cells and other types of macromolecular reactions on the cell surface, as indicated by our preliminary results on the enhancement of antibody binding to cell surfaces ( Supplementary Fig. 8A,B ). Table 1 Enzymatic generation of universal donor red blood cells facilitated by macromolecular crowding. Full size table Using a combination of techniques, insights have been obtained into the mechanisms by which these enzymatic rates are increased on the cell surface in the presence of macromolecular crowders. The increase in enzyme activity in the presence of various polymers is fully consistent with the increased volume exclusion, as the more volume excluded, the higher the effective enzyme concentration. This results in substantial accumulation of enzyme near the cell surface, close to which the polymer crowders cannot approach, as was visualized using fluorescent fusions of the enzyme. Indeed, the cell surface concentration was shown to increase in direct proportion to the polymer concentration. Association of the enzyme with the cell surface will also be enhanced by the interaction of its active site with the cell surface, although clearly from the images measured in PBS this interaction is not of high-enough affinity to saturate the surface in the system under study. Nonetheless, the enzyme remains mobile on the surface, as monitored by FRAP, although increasing crowder concentrations decrease that mobility. This mobility is most probably achieved through a ‘hopping’ mechanism in which enzyme releases from the surface and diffuses to sites nearby, as revealed by exchange experiments using a differently coloured fluorescent fusion partner. Such a model then probably explains a further source of the rate enhancements observed, as the released enzyme is largely confined by the crowder to a layer very close to the surface; thus, rebinding of the enzyme is a rapid event. In this way the enzyme can ‘graze’ over the cell surface without substantial loss to bulk solution, thereby largely restricting its diffusion to two dimensions. Although these experiments provide evidence for some of the major contributing factors to rate enhancement, other factors should also be considered. The higher cell surface activity enhancement seen with glycosidases compared with antibody binding possibly relates to the necessarily more dynamic nature of enzyme binding to cell-surface substrates (carbohydrate antigens in this case). Enzymes modify their binding ligand thus must move as they cleave, whereas antibodies can simply rebind at the same site. Differences between glycosidases could be due to variations in their interactions with cell-surface carbohydrates, differences in diffusion coefficients and possibly changes in the glycocalyx and the accessibility of sugar antigens on the cell surface in the presence of high concentrations of crowders. A combination of all these factors probably influences the observed enzymatic reaction rate enhancements on cell surfaces. The observation that the presence of a carbohydrate-binding module makes no difference to cleavage rates in the absence of crowder, but results in enhanced cleavage in its presence is surprising and may indicate that part of the crowding effect lies in different ‘presentation’ of the cell-surface binding ligand to the enzyme, or in changes in the enzyme conformation that alter the relationship of the binding domain to the active site. A further possible factor could be an increase in percentage of productive collisions of the enzyme with the cell surface if the average time for rebinding of the enzyme with the surface is less than the rotational re-orientation time. Irrespective of the mechanism by which these interactions come into play on the cell surface, the utility of the approach is clearly demonstrated by the ability to fully modify RBCs at enzyme concentrations that are orders of magnitude lower than those otherwise needed. Five blood group antigen-cleaving enzymes (EmGH109 from Elizabethkingia miricola , BfGH110A from Bacteriodes fragilis , CpGH98 from Clostridium perfringens , and Sp3GH98 CD and Sp3GH98 FL from Streptococcus pneumonia ) and carboxy-terminally GFP- and CFP-tagged catalytically inactive mutants of Sp3GH98 CD were cloned, overexpressed and purified using procedures detailed in Supplementary Materials and Methods . Enzymatic removal of blood group antigens Whole blood from healthy consenting donors was collected into a citrate Vacutainer using a protocol approved by the clinical ethics committee of the University of British Columbia. The tube was spun at 1,000 g for 4 min, RBCs were separated and washed three times with PBS buffer (pH 7.4). Washed RBCs (400 μl, 10% haematocrit) were placed in an eppendorf tube, the supernatant was partially removed and replaced with crowder solutions at concentrations from 25 to 300 mg ml −1 . RBCs were mixed carefully and placed on an orbital shaker for 30 min. Diluted enzyme solutions were then added to a final volume of 400 μl. In the case of EmGH109, for example, the concentration of enzyme ranged from 0.4 to 30 nmol ml −1 . The tubes were vortexed very gently and placed on an orbital shaker for 1 h at room temperature (22 °C). After reaction, RBCs were washed three times with an excess of saline and used for analysis. Haemagglutination plate evaluation of cell-surface antigen removal Enzymatically treated, washed RBCs (100 μl, 5% haematocrit) were placed on a haemagglutination plate (Canadian Blood Service, P/N—J028183). Ten microlitres of murine monoclonal antibodies (Dominion Biologicals Limited, Nova Scotia, Canada, catalogue numbers 5170 for anti-A and 5175 for anti-B) was added as a separate drop beside the RBCs (yellow drops in Supplementary Fig. 1A ). RBCs were mixed with antibody by manually flipping the plate, and agglutination time was determined visually when small aggregates of blood were formed: images of the RBCs were taken at different time points ( Supplementary Fig. 1B ). The experiment was conducted for 30 min to minimize the impact of water evaporation on experimental results. Polymeric macromolecular crowders used in this study include dextran and ficoll (Amersham Pharmacia Biotech AB, Sweden), PEG and PVP (Sigma Aldrich, Canada), and HPG that was prepared in the lab using the ring opening multibranching anionic polymerization of glycidol [51] , [52] , [53] . PVP was dialysed using 1 kDa molecular cutoff cellulose ester dialysis membrane (Spectra/Por Biotech, USA) for 3 days and freeze dried before use. Dextran and ficoll were used as received. Micro typing system cards RBCs (12 μl, 5% haematocrit), suspended in diluent (MTS, Florida, USA), were added carefully to the mini gel column, leaving a space between the blood and the contents of the mini gel. The MTS cards were centrifuged at 156 g for 6 min using a Beckman Coulter Allegra X-22R centrifuge with a modified sample holder as recommended. The extent of antigen removal from the surface of the RBC was evaluated from the location of RBCs in the mini gel after spinning according to the manufacturer’s instructions. RBCs with a high surface antigen concentration (for example, positive control) agglutinated on interaction with the monoclonal antibody present in the gel column and could not penetrate (score +4 in Supplementary Fig. 1D ). RBCs with no surface antigens (negative control and RBCs from which surface antigens have been completely removed) did not agglutinate and migrated to the bottom of the mini gel (score 0 in Supplementary Fig. 1C,D ). RBCs that underwent partial removal of surface antigens migrated to positions between these and were assigned scores between 0 and 4 according to the manufacturer’s instructions. Flow cytometry analysis The extent of antibody binding to surface proteins in the presence of different crowders and at different crowder concentrations was determined through flow cytometry analysis, using fluorescently labelled antibodies. Rhesus D antigen analysis RBCs (100 μl, 1% haematocrit) were spun at 1,000 g for 2 min. The supernatant was removed partially and replaced with different volumes of crowding solutions (100–300 mg ml −1 ) to a final volume of 100 μl. FITC-labelled mouse anti-human Rhesus D (5 μl, 0.5% BSA, pH 7.4) obtained from Quotient Biodiagnostics, PA, USA, catalogue number (Z499U) was added to the RBC suspension and mixed carefully. The mixture was incubated at RT for 30 min in the dark. RBCs were washed three times with saline, the supernatant was removed and then RBCs were dispersed in PBS buffer (0.75 ml). The suspension was passed through a 25 G5/8 needle to minimize cell clumping and analysed using a BD FACS Canto II flow cytometer acquiring 10,000 events using medium flow. CD 47 cell surface protein analysis RBCs (100 μl, 1% haematocrit) were spun at 1,000 g for 2 min. The supernatant was partially removed and replaced with different volumes of crowding solutions (100–300 mg m −1 ) to a final volume of 100 μl. Phycoerythin mouse anti human CD47 (5 μl, 1/10 dilution, 0.5% BSA, pH 7.4) obtained from BD Pharmingen, CA, USA, catalogue number (556046) was added to the RBC suspension and mixed carefully. The mixture was incubated at RT for 30 min in the dark. RBCs were washed three times with saline, the supernatant was removed and RBCs were located in PBS buffer (0.75 ml), the suspension was passed through a 25 G5/8 needle to minimize cell clumping and analysed using a BD FACS Canto II flow cytometer acquiring 10,000 events using medium flow. Osmotic fragility haemolysis and optical microscopy To evaluate the impact of enzymatic conversion of RBCs in crowded conditions on their structural and functional integrity, enzymatically treated RBCs were washed three times with saline supplemented with 10% plasma. After washing, cells were stored at 40% haematocrit in 1.5 ml eppendorf tubes at 4 °C supplemented with 10% plasma and 25% SAGM (sodium chloride, adenine, glucose and mannitol) solution, according to storage procedures adopted from the Canadian Blood Services. To evaluate the osmotic fragility, enzymatically converted RBCs were treated with different concentrations of saline for 1 h at room temperature and cell lysis was measured using Drabkin’s reagent according to a previously published detailed procedure [51] . The osmotic fragility curves of RBCs enzymatically treated in the presence of crowders were similar to control cells suggesting no membrane damage ( Supplementary Figs 9B, 10A and 11A ). The amount of haemolysis in enzymatically treated RBCs was measured from the amount of haemoglobin in RBC suspension and in supernatant immediately after the treatment and after 1 day of storage using Drabkin’s reagent according to a previously published detailed procedure [51] . The amount of haemolysis in enzymatically treated RBCs in crowded conditions remained below the transfusion threshold of 1%, determined by FDA transfusion safety criteria [54] , [55] (see Supplementary Figs 10B and 11B ). For optical microscopy experiments, enzymatically treated RBCs (50 μl, 5% haematocrit) in the presence of different crowders were washed and located in an eppendorf tube and mixed with anti A or anti B (15 μl) and placed on an orbital shaker at room temperature (22 °C) for 30 min. For optical microscopy analysis, 2 μl of RBC/antibody suspension was located on a microscope glass slide, covered with a cover slip and analysed using a Zeiss Axioskop 2 Plus microscope. Cholesterol content To measure the amount of cholesterol in the membrane of RBCs, enzymatically treated packed RBCs (1 ml) were transferred and mixed with 1 ml of distilled water located in 50 ml Beckman centrifuge tube. Isopropanol (11 ml, from Sigma, Canada) was pipetted slowly into the cell mixture while the suspension is being mixed with a magnetic stirrer. After 2 h, chloroform (7 ml, from Fisher, Canada) was added and the suspension was mixed for an additional 2 h. The tube was centrifuged at 3,000 g for 5 min, the supernatant was removed and filtered through a disposable polypropylene filter (13 mm, from Whatman, UK), the solvent was evaporated overnight, the remaining solid residue was dissolved in glacial acetic acid (3 ml, Fisher, Canada) and the content of cholesterol was determined using the Zlatkis method [56] . The total amount of cholesterol was ~0.88 mg ml −1 of packed RBCs and it was comparable to values reported in the literature [57] . The total amount of cholesterol did not change as a result of enzymatic removal of antigenic carbohydrates from cell surfaces in crowded conditions in 40 kDa dextran (300 mg ml −1 ; see Supplementary Fig. 10 ). Mean corpuscular volume and haemoglobin content The mean corpuscular volume and mean corpuscular haemoglobin content of enzymatically treated RBCs were determined using the automated ADVIA 120 Hematology System (Siemens, Germany). The amounts of mean corpuscular volume and mean corpuscular haemoglobin content of enzymatically treated RBCs in crowded conditions were within the normal range of RBCs determined by the manufacturers’ of ADVIA 120 Hematology System (see Supplementary Figs 10 and 11 ). Removal of sialic acid from RBC surfaces Sialic acid was removed from RBC surfaces using neuraminidase from Clostridium Perfringens (Sigma Aldrich, Canada). RBCs were washed as before and suspended in PBS buffer at pH 6 (400 μl, 10% haematocrit). The supernatant was replaced with different crowder solutions and vortexed, neuraminidase (30 μl, 0.1 U ml −1 ) was added to a final volume of 400 μl. Crowder concentration was varied (0–300 mg ml −1 ) and the impact of crowding on removal of sialic acid from the cell surface was investigated by measuring the cell electrophoretic mobility [49] using the Rank Brothers Mark I Electrophoretic mobility apparatus (Rank Brothers, Bottisham, UK). A drop of 10% haematocrit of RBC was diluted in 10 ml saline (154 mM, pH 7.4) and the velocity of individual cells located in the stationary region was measured at a constant potential. At least ten individual cells were selected randomly and their velocity was measured; results were presented as the mean±s.d. Enzymatic generation of universal blood donor cells The enzymatic conversion of RBCs from at least ten donors with different blood groups such as A + , B + , AB + and B − were investigated in crowded conditions. The ‘+’ and ‘−’ indicate the presence of Rh factor on RBCs. Enzymatically converted and washed RBCs were analysed using FDA-approved MTS cards as explained previously. For the enzymatic conversion of AB group, washed RBCs (400 μl, 10% haematocrit) were placed in an eppendorf tube, the supernatant was partially removed and replaced with 40 kDa dextran solution to a final concentration of 300 mg ml −1 . RBCs were mixed carefully and placed on an orbital shaker for 30 min. To remove A antigens, a diluted EmGH109 enzyme solution was added to a final concentration of 1 nmol ml −1 and volume of 400 μl. The tubes were vortexed very gently and placed on an orbital shaker for 1 h at room temperature (22 °C). After reaction, RBCs were washed three times with an excess of saline. In the case of EmGH109, for example, the concentration of enzyme ranged from 0.4 to 30 nmol ml −1 and used for analysis. To remove B antigens, supernatant was partially replaced with 40 kDa dextran solution as before and diluted Sp3GH98 CD enzyme solution was added to a final concentration of 0.057 nmol ml −1 and volume of 400 μl. The tubes were vortexed gently and placed on an orbital shaker for 1 h at room temperature (22 °C). After reaction, RBCs were washed three times with an excess of saline and analysed (see Supplementary Fig. 9A ). Polymer hydration measurements The amount of free water associated with macromolecular crowder at different concentrations was determined from the ratio of the enthalpy of fusion of free water in the polymer solution to the ratio of the enthalpy of a similar weight of pure water using a Q 2100 differential scanning calorimetry from TA Instruments [51] . Briefly, around 20 μl of crowder solution was heated at a rate of 0.2 °C min −1 after cooling rapidly to −30 °C and the fusion enthalpy was measured using the TA analysis software. HPG (10, 30 and 110 kDa), dextran (10, 40 and 110 kDa) and ficoll (70 kDa) were used. Three different concentrations were tested 10, 20 and 30 w/w%. Immobilization of RBCs onto the glass surface RBCs were immobilized on the glass surface, as cells otherwise floated in the presence of high crowder concentrations, interfering with fluorescence intensity measurements due to Brownian motion. A confocal quality glass surface attached to the bottom of a petri dish obtained from Willco Wells (Amsterdam, The Netherlands) was treated with detergent (10% Extran solution) for 2 h. After rinsing with distilled deionized water, poly- L -lysine solution (300 μl of 0.01%, molecular weight=70,000–150,000 Da, Sigma, ON, Canada) was added and left for 1 h. Polymer solution was removed, the glass was rinsed and a glutaraldehyde solution (300 μl of 1%, Sigma) was added and left for 10 min. The glass surface was rinsed with distilled water followed by rinsing with PBS pH 7.4. RBCs (300 μl, 4% haematocrit) were added and incubated at room temperature (22 °C) for 10 min. Supernatant was then pipetted out and non-bound blood was removed by rinsing with PBS. PBS solutions (200 μl) supplemented with different crowders at a range of concentrations were added carefully and images collected using the Nikon C2+ Eclipse Ti-E confocal microscopy. The concentration of GFP-Sp3GH98 E558A CD enzyme was 1.3 nmol ml −1 and that of the crowders was between 0 and 320 mg ml −1 . The concentration of enzyme was optimized to obtain clear fluorescent images using low laser powers. Immobilization of GFP-Sp3GH98 E558A CD on cell surface GFP-Sp3GH98 E558A CD was immobilized on the cell surface using a glutaraldehyde solution (Grade II 25% in water, obtained from Sigma Aldrich). Glutaraldehyde solution was added to PBS containing different concentrations of dextran 40 kDa (90–320 mg ml −1 ), after which GFP-Sp3GH98 E558A CD enzyme was added and the mixture (200 μl) placed on the surface of cells immobilized on glass slides. The mixture was equilibrated for 3 h at room temperature (22 °C) before imaging. The concentration of glutaraldehyde was 6% and GFP-Sp3GH98 E558A CD was 1.3 nmol ml −1 . Fluorescence recovery after photobleaching FRAP experiments were carried out using a × 60 oil immersion objective at room temperature (22 °C). A circular region with a radius of 5.5 μm on the cell surface was bleached for 1.95 s using a laser intensity that ranged from 40 to 60% of the maximum laser power at 488 nm (11 mW), after which the fluorescence recovery was recorded for around 300 s. The diffusion coefficient was calculated using equation (1) given by Axelrod et al . [41] , where w is the half-width at 1/ e 2 height of the Gaussian profile of the bleached spot intensity [41] , is the characteristic diffusion time that was determined by fitting equation (2) to fluorescence recovery curve of the mobile fraction of the diffusing enzyme. K is the bleaching constant that was determined from the following equation [41] , [43] : where is the fluorescence intensity of the bleached spot immediately after bleaching and is the fluorescence intensity of the bleached spot before bleaching. The mobile fraction of the enzyme was determined from equation (4) given by Blonk et al . [41] : where and is the fluorescence intensity of the bleached spot after recovery. In our experiments, was determined from equation (1) using FITC-BSA as a probe according to a procedure adapted from Banks and Fradin [42] . The diffusion coefficient of FITC-BSA ( D FITC-BSA ) was 68 μm 2 s −1 as reported in the literature [45] . The characteristic diffusion time of FITC-BSA was obtained by fitting equation (2) to experimental fluorescence recovery data of FITC-BSA using the least squares fitting, and w was determined from equation (1). The emitted fluorescence in our experiments was focused through a 1.2 AU (30 μm) diameter pinhole. Exchange of enzymes on cell surfaces To evaluate the impact of crowding on the association of enzymes with cell-surface antigens, GFP-labelled (GFP-Sp3GH98 E558A CD, green) mutant enzyme in PBS or crowder (75 μl, 1.3 nmol ml −1 ) was placed initially on the cell surface to associate with cell-surface antigens, after which a layer of CFP-labelled CFP-Sp3GH98 E558A CD( cyan) (75 μl, 10.7 nmol ml −1 was added carefully and the depletion of GFP-Sp3GH98 E558A CD (green) from cell surface and its replacement with CFP-Sp3GH98 E558A CD (cyan) was investigated using confocal microscopy. The fluorescence intensity on the cell surface was measured at different time points using both the green and cyan channels at 488 and 457 nm. The experiments were performed at room temperature (22 °C). Higher concentration of CFP-Sp3GH98 E558A CD, cyan, was used for better visualization of exchange process. To determine the time during which CFP-Sp3GH98 E558A CD diffuses from the top layer through the bottom layer before interacting with GFP-Sp3GH98 E558A CD on the cell surface, a transparent layer of PBS or crowder (75 μl) was added to the cell surface. The transparent layer contained the minimum amount of GFP-Sp3GH98 E558A CD required to focus the cells using the confocal microscope. A layer of GFP-Sp3GH98 E558A CD in PBS or crowder (75 μl, 1.3 nmol ml −1 ) was pipetted carefully on top of the transparent layer and the fluorescence intensity of the green channel at 488 was acquired at different time points. The per cent of enzyme that had diffused to the cell surface was determined from the ratio of fluorescence intensity to equilibrated fluorescence intensity 3 h after the addition of the top layer. The fluorescence intensity distribution of glass attached cells at different locations was investigated by acquiring z -stack images of cells using a total thickness of 10 μm with 0.2 μm intervals. Two fluorescent peaks were observed, a sharp peak attributed to enzyme present on the glass surface and a wider peak attributed to enzyme present on the cell surface ( Supplementary Fig. 5B,C ). Statistics All data are presented as a mean±s.d. unless otherwise mentioned. Where indicated, one-way analysis of variance test was performed using Origin 7.0. Paired comparisons were considered to be significant when P <0.05. How to cite this article: Chapanian, R. et al . Enhancement of biological reactions on cell surfaces via macromolecular crowding. Nat. Commun. 5:4683 doi: 10.1038/ncomms5683 (2014).